Multiplexed volumetric bar-chart chip for point-of-care diagnostics Microfluidics have become an enabling technology for point-of-care and personalized diagnostics. Desirable capabilities of microfluidics-based diagnostic devices include simplicity, portability, low cost and the performance of multiplexed and quantitative measurements, ideally in a high-throughput format. Here we present the multiplexed volumetric bar-chart chip (V-Chip), which integrates all these capabilities in one device. A key feature of the V-Chip is that quantitative results are displayed as bar charts directly on the device—without the need for optical instruments or any data processing or plotting steps. This is achieved by directly linking oxygen production by catalase, which is proportional to the concentration of the analyte, with the displacement of ink along channels on the device. We demonstrate the rapid quantification of protein biomarkers in diverse clinical samples with the V-Chip. The development of the V-Chip thus opens up the possibility of greatly simplified point-of-care and personalized diagnostics. Major technological challenges remain in the development of personalized diagnostics, including improvements of assay throughput and time, reductions in operating costs and training, and optimization of equipment portability and accessibility [1] , [2] , [3] . Over the past decade, microfluidics-based point-of-care (POC) diagnostics have been developed to meet such challenges [4] . In principle, because of the high degree of integration of fluidic handling, specimen processing and consumption of reagents, microfluidic-based POC platforms can perform quantitative, rapid and affordable high-throughput measurements, and therefore have the potential to revolutionize clinical genomic and proteomic analyses and personalized diagnostics [5] , [6] . However, in practice, several problems are usually encountered. First, the fluid-introducing accessories and pump control systems in microfluidics platforms result in significant additional cost and operational space [7] ; second, the collection of assay results still requires traditional instruments, such as fluorescence, absorption, or mass spectrometers, electrochemical or glucose metres, and others [7] , [8] , [9] , [10] , [11] ; and third, complicated fluidic networks limit the number of measurements per chip and thereby throughput of the device. These practical barriers limit the application of microfluidic chips in clinics and in patients’ homes. The integration of an on-chip mechanical pump has minimized accessory requirements; that is, replacing the large pressure system with a battery or an on-chip power supply [12] , [13] , [14] ; SlipChip technology, allowing the breaking or connexion of flow paths through hand-movements of glass plates instead of switching microfluidics valves, has simplified fluidic handling and removed the need for pump accessories [15] , [16] ; and paper-based microfluidics devices discard pressurized flow and use capillary force, which also improves the portability of the device [17] , [18] . All of these developments have succeeded in reducing device size and operational complexity and represent a start towards solving the first challenge listed above. The second and third challenges, however, remain major barriers for microfluidic-based POC applications. Herein, we report the development of a new device, the multiplexed volumetric bar-chart chip (V-Chip) that can meet all three challenges. Instead of using chemiluminescence or fluorescence readouts, the V-Chip presents an on-chip visualized bar chart, based on the volumetric measurement of oxygen generation on-chip, integrated with an enzyme-linked immunosorbent assay (ELISA) reaction ( Fig. 1 ). The design employs catalase as the ELISA probe, which is conjugated to silica nanoparticles functionalized with ELISA detection antibodies. Catalase reacts with hydrogen peroxide to release oxygen. The reaction is very sensitive and activated within seconds after the two agents are brought in contact with each other [19] . The generated oxygen accumulates within the limited volume of the microfluidics channels and causes an increase in pressure, which pushes preloaded inked bars ( Fig. 1a ). The advancement of each individual inked bar independently indicates the amount of catalase that reacted in that ELISA well, which correlates with the concentration of the corresponding ELISA target [19] . This approach allows for the measurement of target protein biomarkers in both a quantitative and multiplexed manner. 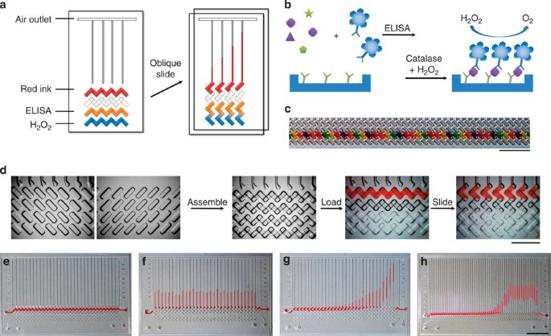Figure 1: Working principle of the V-Chip. (a) Schematic view of a typical V-Chip. On the left is a view of an assembled V-Chip with the flow path at the horizontal position. Ink and H2O2can be preloaded and the ELISA assay can be performed in the designated lanes. An oblique slide breaks the flow path and forms the structure on the right, causing catalase and H2O2to react and push the inked bars. (b) V-Chip ELISA reaction scheme and the oxygen generation mechanism. (c) Image of 50 sample wells loaded with different coloured food dyes using swab tips. Scale bar, 0.5 cm. (d) Zoomed microscopic images of as-fabricated bottom and top plates, device assembly, reagent loading and assay operation in a 50-plexed V-Chip. Scale bar, 2.5 mm. (e) A 30-plexed V-Chip loaded with the red ink and reagents. (f) Uniform ink advancement image resulting from the application of equal concentrations of catalase. (g,h) Progressive ink advancement in 30- and 50-channel V-Chips generated by the 3- and 6-h diffusion of catalase from the drilled holes on the right to the ELISA lane at room temperature. Scale bar, 1 cm ine,f,gandh. Figure 1: Working principle of the V-Chip. ( a ) Schematic view of a typical V-Chip. On the left is a view of an assembled V-Chip with the flow path at the horizontal position. Ink and H 2 O 2 can be preloaded and the ELISA assay can be performed in the designated lanes. An oblique slide breaks the flow path and forms the structure on the right, causing catalase and H 2 O 2 to react and push the inked bars. ( b ) V-Chip ELISA reaction scheme and the oxygen generation mechanism. ( c ) Image of 50 sample wells loaded with different coloured food dyes using swab tips. Scale bar, 0.5 cm. ( d ) Zoomed microscopic images of as-fabricated bottom and top plates, device assembly, reagent loading and assay operation in a 50-plexed V-Chip. Scale bar, 2.5 mm. ( e ) A 30-plexed V-Chip loaded with the red ink and reagents. ( f ) Uniform ink advancement image resulting from the application of equal concentrations of catalase. ( g , h ) Progressive ink advancement in 30- and 50-channel V-Chips generated by the 3- and 6-h diffusion of catalase from the drilled holes on the right to the ELISA lane at room temperature. Scale bar, 1 cm in e , f , g and h . Full size image Design and fabrication of the V-Chip The V-Chip employs SlipChip technology [15] , [16] but introduces new flow paths and a new readout strategy. In the SlipChip, two pieces of glass etched with microfluidic wells and channels are assembled together in the presence of mineral oil. A fluidic path is formed when the two plates aligned in a specific configuration. Samples or reagents are preloaded through drilled holes using a pipette, and the top plate is then moved relative to the bottom plate to enable the diffusion and reaction of samples or reagents. Unlike previous SlipChip methods, our V-Chip employs catalase as a probe to generate oxygen, directly linking the ELISA reaction to the generation of ink-based bar charts and the direct visualization of assay results without the need for external instruments. Two 75 × 50-mm glass slides are used to fabricate the V-Chip device. Channel patterns are first drawn with AutoCAD software and fabricated onto glass surfaces by standard photolithography and glass etching methods. A detailed protocol is provided in the Methods section and in Supplementary Fig. S1 . Typical finished top and bottom plates are shown in Supplementary Fig. S2 . We have designed and fabricated devices with different throughput levels, including single-, 6-, 10-, 30- and 50-plexed measurements. Working principle of the V-Chip As shown in Fig. 1a , the device is first placed in the loading position after assembly, where the rectangular wells of the top plate and the bottom plate partially overlap to form an ‘N’-shaped fluidic path from the left side to the right side in the horizontal direction. In this position, reagents or samples can be loaded through the drilled holes on the left of the V-Chip ( Supplementary Fig. S2 ). Before the sample assay, the top flow lane is preloaded with ink and the second lane from the top is kept blank to serve as an air spacer, thereby avoiding direct contact between the sample and the ink. This is essential because hydrogen peroxide may bleach the ink solution and affect the visual readout of the results. The third lane is the sample lane, where the ELISA assay is carried out. This lane can also be filled with catalase molecules directly for an oxygen generation test. The bottom-most lane is preloaded with hydrogen peroxide. An oblique slide of the device causes the horizontal fluidic paths to separate and re-form into independent units arranged in parallel in the vertical direction ( Fig. 1a and Supplementary Movie 1 ). In each vertical unit, the wells partially overlap to form a closed ‘Z’-shaped path, bringing the hydrogen peroxide into contact with the catalase probe. Instantly, oxygen is generated and the ink in the top row of wells is pushed into the small bars ( Fig. 1a and Supplementary Movie 2 ). Because the channels are vented to atmospheric pressure, the ink bands will continue moving in the channel until the oxygen produced is insufficient to push them. To stop the movement of the ink bar for a stable reading, the glass plates can be slipped back to the original loading position, releasing the generated oxygen through the loading holes and thereby discontinuing the propulsion of the inked bars. Sliding back the glass plates separates the vertical connexions and thereby immediately stops the ink movement. The oxygen, which is released in the horizontal direction, will not cause a spill-out as the inlet/outlet holes can serve as reagent reservoirs. Validation and optimization of V-Chip ELISA assays Before the V-Chip ELISA assay, capture antibodies are covalently immobilized on the epoxy-terminated glass surface in the sample wells ( Fig. 1b and Supplementary Fig. S3 ; [20] ). Coating with multiple capture antibodies can be achieved by microarray printing or simply by inking the wells with a sharp swab tip ( Fig. 1c ). The roughness of the etched glass surface in the capture antibody wells greatly increases the coating efficiency ( Supplementary Fig. S4 ). The location of the capture antibody and the multi-well surface coating are demonstrated in Fig. 1c , in which food dyes are used to visually represent each individual antibody. After the assembly of the V-Chip, an assay sample (for example, cell lysate or patient serum) is flowed through the ELISA channel (the third lane of the V-Chip fluidic handling region). Because of the ultra-miniaturization in microfabrication technology, only a 10-μl sample is required to complete a V-Chip ELISA reaction to detect biomarkers in serum. This is a great advantage for the application of the device to a POC blood test, for which a finger prick might be sufficient and invasiveness can be dramatically reduced. After the protein targets are captured by the V-Chip ELISA chambers via specific antibody–antigen reactions, a mixture of all the catalase-detecting probes (silica nanoparticles conjugated with detecting antibodies and catalase molecules) is applied. Each reaction well will form an independent sandwich structure in which its specific target antigen is captured. Repeated washing steps are applied to reduce the nonspecific binding in the V-Chip assay. Our scanning electron microscope (SEM) images indicate that the catalase probes efficiently bind onto the glass surface in the presence of antigen targets ( Supplementary Fig. S5 ). At this stage, all protein targets and their corresponding amounts of catalase probes are positioned in individual wells and will not move even when V-Chip flow paths change from the ‘N’ to the ‘Z’ shape. At the readout position, the ‘Z’-shaped flow path allows the catalase probe to make contact with hydrogen peroxide, producing oxygen, which triggers the immediate movement of the inked bars. The volume of oxygen generated correlates with the amount of catalase and the target concentration; the design is therefore able to quantitate proteins based on the advancement of the inked bars. Figure 1d shows the assembly, reagent loading and slide operation of a 50-plex V-Chip. The top plates and the bottom plates were aligned and partly overlapped to form the ‘N’ shaped lanes. During device assembly, fluorinated oil was used as a lubricant and to render the device airtight. Following sample loading, an oblique slide separated the horizontal fluidic paths and the wells re-connected in the vertical direction ( Fig. 1d ). In this position, the wells containing hydrogen peroxide and the wells containing catalase overlapped partially, allowing the hydrogen peroxide solution to diffuse and react with catalase. To demonstrate that ink movement is related to catalase concentration, catalase solutions were directly loaded through the drilled holes in the V-Chip for an oxygen generation test. Figure 1e shows a 30-plex V-Chip that was loaded with reagents and samples. When a uniform catalase concentration was applied to the V-Chip, the bar charts showed uniform advancement ( Fig. 1f ); whereas with a gradient of catalase, created by a 3-h diffusion of catalase from an inlet on the bottom-right of the device, the frontier of the bar chart resembled a sigmoidal shape ( Fig. 1g ; [21] ). Figure 1h demonstrated another sigmoidal bar chart advancement pattern in a 50-plex V-Chip with a 6-h diffusion of catalase. The progressive increments indicate that the distance moved by each ink bar correlates to the concentration of the diffused catalase. The data shown in Fig. 1f–h clearly demonstrate the relationship between the advancement of the V-Chip bars and the catalase concentration. One of the key requirements for POC assays is a timely and quantitative readout. Several factors may impact the V-Chip readout, including the amount of catalase, hydrogen peroxide concentration, reaction temperature and assay time. To optimize the assay, we prepared a single-channel V-Chip and tested all the above-listed conditions ( Fig. 2 ). As shown in Fig. 2a , we directly loaded catalase molecules at concentrations ranging from 3 to 30 U into the top chamber, and loaded hydrogen peroxide at a concentration of 0.45 M to the bottom chamber. Upon vertically sliding the V-Chip, the catalase molecules were brought into contact with hydrogen peroxide and oxygen was immediately produced, causing the red ink in the centre of the V-Chip to be pushed to the readout region. The movements of the ink were recorded as movies and the time dependence of ink advancement is plotted in Fig. 2c . The rate of ink movement was positively correlated with catalase concentration, and a pseudo-linear relationship between catalase concentration and ink movement distance was observed at 1, 2 and 6 min ( Fig. 2d ). All three intervals show appropriate linearity; however, more discriminable ink distances are present in intervals larger than 2 min. We maintained a consistent readout time for each batch of experiments to achieve comparable quantitation. 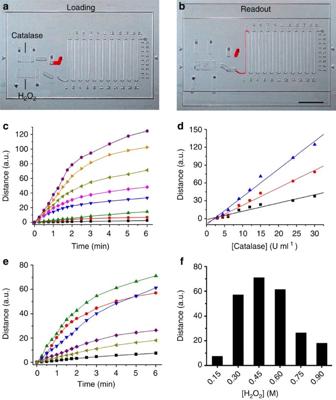Figure 2: Assays using a single-channel V-Chip. (a) In the loading position of the chip, H2O2, catalase and ink are loaded in the indicated wells. (b) Ink advancement in the V-Chip is pushed by oxygen generated as a result of catalase reacting with H2O2. Scale bar, 1 cm for bothaandb. (c) Time-dependent ink advancement with the application of different concentrations of catalase and 0.45 M H2O2, at room temperature. The concentrations of catalase used were 3 U ml−1(black), 4.5 U ml−1(red), 6 U ml−1(green), 9 U ml−1(blue), 12 U ml−1(magenta), 15 U ml−1(brown-green), 24 U ml−1(orange) and 30 U ml−1(purple). (d) Linearity curves of the ink advancement readout, with different catalase concentrations and in different time ranges: 1 min (black), 2 min (red) and 6 min (blue). (e) Time-dependent ink advancement with the application of different concentrations of H2O2and 15 U catalase, at room temperature. The concentrations of H2O2used were 0.15 M (black), 0.3 M (red), 0.45 M (green), 0.6 M (blue), 0.75 M (purple) and 0.9 M (brown-green). (f) Ink advancement after 6 min plotted against H2O2concentration. Figure 2: Assays using a single-channel V-Chip. ( a ) In the loading position of the chip, H 2 O 2 , catalase and ink are loaded in the indicated wells. ( b ) Ink advancement in the V-Chip is pushed by oxygen generated as a result of catalase reacting with H 2 O 2 . Scale bar, 1 cm for both a and b . ( c ) Time-dependent ink advancement with the application of different concentrations of catalase and 0.45 M H 2 O 2 , at room temperature. The concentrations of catalase used were 3 U ml −1 (black), 4.5 U ml −1 (red), 6 U ml −1 (green), 9 U ml −1 (blue), 12 U ml −1 (magenta), 15 U ml −1 (brown-green), 24 U ml −1 (orange) and 30 U ml −1 (purple). ( d ) Linearity curves of the ink advancement readout, with different catalase concentrations and in different time ranges: 1 min (black), 2 min (red) and 6 min (blue). ( e ) Time-dependent ink advancement with the application of different concentrations of H 2 O 2 and 15 U catalase, at room temperature. The concentrations of H 2 O 2 used were 0.15 M (black), 0.3 M (red), 0.45 M (green), 0.6 M (blue), 0.75 M (purple) and 0.9 M (brown-green). ( f ) Ink advancement after 6 min plotted against H 2 O 2 concentration. Full size image We also optimized the hydrogen peroxide concentration using a similar strategy ( Fig. 2e ). Surprisingly, the highest hydrogen peroxide concentration did not provide the furthest ink advancement, because catalase activity was inhibited when the hydrogen peroxide concentration reached a certain threshold [19] . On the basis of the results shown in Fig. 2f , the optimum hydrogen peroxide concentration was identified as 0.45 M for 15 U catalase at room temperature. In the absence of catalase, 0.45 M hydrogen peroxide decomposes very slowly and the generated oxygen is not able to move the inked bars. Storing the loaded device in the dark can further reduce the hydrogen peroxide decomposition. Catalase activity is also related to reaction temperature, but the assay works at both room temperature and 37 °C. We observed that the movement of the red ink band was slightly faster at 37 °C than at room temperature ( Supplementary Fig. S6 ). However, consistent temperature control is more difficult at 37 °C than at room temperature. To reduce the complexity and cost for POC applications, the experiment was performed at room temperature (25 °C). During the operation, the operator’s fingers should avoid touching the catalase reaction zone to minimize temperature changes. On the basis of the results of the assay-optimizing experiments shown in Fig. 2 , we identified the ideal reaction conditions: a hydrogen peroxide concentration of 0.45 M, reaction at room temperature, and a time interval of 2–6 min for the readout. Single-channel V-Chip ELISA assay We first tested the ELISA reaction with a human chorionic gonadotropin (hCG) protein target using a single-channel V-Chip. hCG is a pregnancy indicator and widely accepted biomarker for some types of cancer, including breast and ovarian cancer [22] . We prepared a single-channel V-Chip and performed repeated hCG assays using the same chip. To conveniently reuse the V-Chip, we used 2.8-μm magnetic beads conjugated with the hCG capture antibody for the ELISA reaction. The beads were held at the bottom of the ELISA well by a magnet ( Fig. 3a ) and replaced with new particles for a new assay with a different hCG concentration. We tested a range of hCG concentrations from 2 to 1 × 10 5 mIU and compared the assay results with a commercially available pregnancy test. 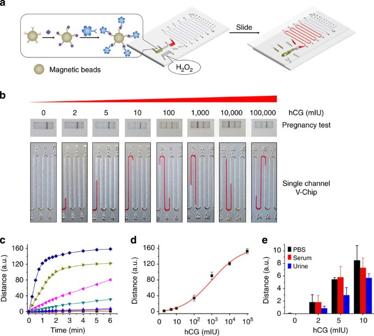Figure 3: Detection of hCG using a single-channel V-Chip. (a) V-Chip hCG detection scheme. In the ELISA well, hCG is captured by magnetic beads functionalized with capture antibodies, and detected by catalase-conjugated silica nanoparticles functionalized with detecting antibodies. The reaction is initiated by sliding the V-Chip. (b) Comparison of the commercial pregnancy test and the V-Chip for sensing hCG in PBS buffer. (c) Time-dependent ink advancement in the presence of different concentrations of hCG: 2 mIU (black), 5 mIU (red), 10 mIU (blue), 1 × 102mIU (cyan), 1 × 103mIU (magenta), 1 × 104mIU (brown) and 1 × 105mIU (navy). (d) The hCG calibration curve corresponding to ink advancement at 6 min, with the hCG concentration varying from 2 mIU to 1 × 105mIU. (e) Detection results of spiked hCG in PBS buffer, serum and urine. The error bars indanderepresent the s.d. of three measurements. Figure 3b presents the back-to-back 6-min assay results from the pregnancy kit and the V-Chip test. At low hCG concentrations, the pregnancy kit result showed a weak signal at 5 mIU and no signal at 2 mIU, while the V-Chip presented clear ink advancement even at the 2 mIU hCG concentration. At high concentrations, because of the hook effect [23] , the pregnancy test kit began to lose signal due to the binding saturation by the extra amount of the target, while the V-Chip still presented visual and quantitative results. Over the entire hCG concentration range, the V-Chip was able to visualize and quantify the target ( Fig. 3c ). The V-Chip also works with more complex sample matrices, such as serum and urine ( Fig. 3e ). Figure 3: Detection of hCG using a single-channel V-Chip. ( a ) V-Chip hCG detection scheme. In the ELISA well, hCG is captured by magnetic beads functionalized with capture antibodies, and detected by catalase-conjugated silica nanoparticles functionalized with detecting antibodies. The reaction is initiated by sliding the V-Chip. ( b ) Comparison of the commercial pregnancy test and the V-Chip for sensing hCG in PBS buffer. ( c ) Time-dependent ink advancement in the presence of different concentrations of hCG: 2 mIU (black), 5 mIU (red), 10 mIU (blue), 1 × 10 2 mIU (cyan), 1 × 10 3 mIU (magenta), 1 × 10 4 mIU (brown) and 1 × 10 5 mIU (navy). ( d ) The hCG calibration curve corresponding to ink advancement at 6 min, with the hCG concentration varying from 2 mIU to 1 × 10 5 mIU. ( e ) Detection results of spiked hCG in PBS buffer, serum and urine. The error bars in d and e represent the s.d. of three measurements. Full size image Multiplexed V-Chip ELISA assay A primary concern in cancer diagnosis and prognosis is the correct classification of the patient’s disease stage. The clinical method for the identification and classification of human tumours is mostly based on immunohistochemistry and fluorescence in situ hybridization [24] . ELISA is an alternative [25] that is frequently used in monitoring the response to therapy by measuring tissue lysates and in follow-up care of patients when measuring serum biomarkers. Despite the reduced sensitivity caused by mixed cell populations, ELISA technology is still the only reliable test for large sample sizes that has the quantitative capability to analyse biomarker expression as a continuous variable rather than a dichotomous variable [25] . Therefore, ELISA technology serves as the standard to establish the cutoff point and define biomarker overexpression for the selection of optimal therapy strategies. Most tumours, including breast cancer, are highly heterogeneous [26] . A single biomarker measurement is not reliable for diagnosis or classification. The inclusion of more biomarkers and the use of multiplexed assays are believed to be able to increase accuracy [27] , [28] , [29] ; however, this will increase diagnostic cost significantly. In our multiplexed V-Chip, the micro-sized channels require minimal amounts of reagent and the parallel operation reduces assay time, thereby significantly reducing assay cost compared with traditional diagnostic approaches. In contrast to traditional ELISA methods, the V-Chip device is portable, affordable and potentially user-friendly, which might be suitable for disease monitoring in resource-limited areas such as developing countries or in home blood testing. To demonstrate the multiplexed capability of the V-Chip, we generated a six-plexed chip for breast cancer cell classification. We included the oestrogen receptor (ER), progesterone receptor (PR) and human epidermal growth factor receptor 2 (HER2) biomarkers in the V-Chip, and used the remaining blank bars as controls [30] . To assess whether our device can accomplish ER, PR and HER2 profiling, cells from five breast cancer lines (BT-474, MCF-7, SKBR-3, SUM-159 and MDA-MB-231) were counted, directly lysed in RIPA buffer and used to validate the capability of the V-Chip assay. According to previous reports, ER, PR and HER2 are all overexpressed in BT-474 cell lines ( Fig. 4a ; [30] ). 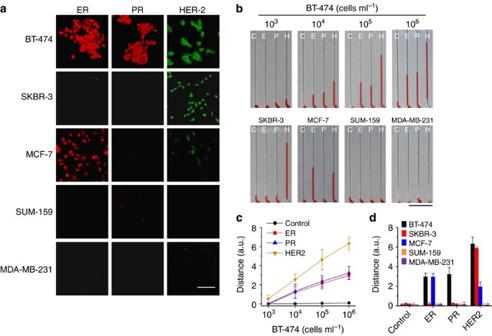Figure 4: Multiplexed detection of biomarkers from cell lysates. (a) Fluorescent images of BT-474, SKBR-3, MCF-7, MDA-MB-231 and SUM-159 cells, stained with Cy3 (ER and PR) and FITC (HER2). Scale bar, 100 μm. (b) The top four ink advancement images show the results of assays on BT-474 lysates with increasing numbers of cells; the bottom four images show the results of the assays on SKBR-3, MCF-7, SUM-159 and MDA-MB-231 cell lysates with a concentration of 1 × 106cells ml−1. C, E, P and H represent control, ER, PR and HER2, respectively. Scale bar, 1 cm. (c) Quantitation curves of ER, PR and HER2 in BT-474 assays. (d) V-Chip readouts of the five cell lysates at a concentration of 1 × 106cells ml−1. The error bars incanddrepresent the s.d. of three measurements. Figure 4b shows the distance moved by the red ink bands in the presence of different amounts of BT-474 cells. As the number of BT-474 cells increased, the bar distance values of the three biomarkers changed accordingly, indicating that ER, PR and HER2 are all expressed in the BT-474 cell line. The control channels never moved a significant distance larger than 0.3 V-Chip unit ( Fig. 4b ). The dependent increment of the distances for ER, PR and HER2 suggests that the V-Chip may be suitable for clinical use to evaluate the levels of these receptors. Using this device, we can detect these biomarkers with sample sizes as low as 1000 BT-474 cells ml −1 ( Fig. 4c ). Figure 4: Multiplexed detection of biomarkers from cell lysates. ( a ) Fluorescent images of BT-474, SKBR-3, MCF-7, MDA-MB-231 and SUM-159 cells, stained with Cy3 (ER and PR) and FITC (HER2). Scale bar, 100 μm. ( b ) The top four ink advancement images show the results of assays on BT-474 lysates with increasing numbers of cells; the bottom four images show the results of the assays on SKBR-3, MCF-7, SUM-159 and MDA-MB-231 cell lysates with a concentration of 1 × 10 6 cells ml −1 . C, E, P and H represent control, ER, PR and HER2, respectively. Scale bar, 1 cm. ( c ) Quantitation curves of ER, PR and HER2 in BT-474 assays. ( d ) V-Chip readouts of the five cell lysates at a concentration of 1 × 10 6 cells ml −1 . The error bars in c and d represent the s.d. of three measurements. Full size image Using a cell concentration of 10 6 cells ml −1 , the V-Chip was next used to distinguish the biomarker expression profiles of different breast cancer cell lines ( Fig. 4b , bottom). Considering the distance values in BT-474 cells to be 100%, and assuming that the distance values are proportional to biomarker expression, SKBR-3 cells expressed 92% HER2, while MCF-7 cells expressed 92% ER and 29% HER2 ( Fig. 4d ). However, these three biomarkers were rarely expressed in SUM-159 and MDA-MB-231 cells, which are known to have low expression of ER, PR and HER2. These results are consistent with previous reports and our own fluorescent measurements [30] . Parallel measurements of multiple serum samples Carcinoembryonic antigen (CEA) has become one of the most convincing serum biomarkers as it provides fast, non-invasive, reproducible and quantitative indications in follow-up care and when monitoring the therapy of breast cancer patients. Although CEA cannot be used to diagnose primary cancer, its applications in early-stage prediction of metastases and in monitoring the response to metastatic therapy are promising [31] . To assess the prognostic value of serum biomarkers, multivariate analysis of a large number of patient sera in a short follow-up period is required [32] . In the present work, we tested serum samples from 10 patients using the V-Chip. 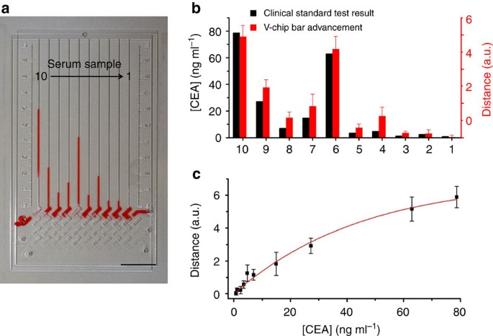Figure 5: V-Chip CEA assays on patient sera. (a) A typical CEA readout of 10 patient sera analysed on the V-Chip. Scale bar, 1 cm. (b) Bar graphs of the CEA concentration measured by the ADVIA Centaur Instrument (black) and the V-Chip distance (red), side-by-side. The error bars represent the s.d. of three V-Chip measurements. (c) Plot of V-Chip bar distances against CEA concentration. The error bars represent the standard deviation of three measurements. Figure 5a shows a V-Chip assay image of the 10-serum test and Fig. 5b shows both the results from the clinical ELISA method ( Supplementary Fig. S7 and Supplementary Table S1 ) and the average bar advancements of three V-Chip tests listed side-by-side. The trends of both types of tests are correlated. In the plot of V-Chip ink advancement against CEA concentration values in Fig. 5c , it is not surprising that the curve is pseudo-exponential rather than linear. The causes may include antibody–antigen binding constant, catalase catalytic activity and other related thermodynamic effects. It should be noted that the sensitivity of the V-Chip is not as good as that of highly sophisticated clinical instruments and that the V-Chip performs better at concentrations higher than 5 ng ml −1 . The sensitivity of the V-Chip can certainly be improved if narrower and longer bar channels are used. Figure 5: V-Chip CEA assays on patient sera. ( a ) A typical CEA readout of 10 patient sera analysed on the V-Chip. Scale bar, 1 cm. ( b ) Bar graphs of the CEA concentration measured by the ADVIA Centaur Instrument (black) and the V-Chip distance (red), side-by-side. The error bars represent the s.d. of three V-Chip measurements. ( c ) Plot of V-Chip bar distances against CEA concentration. The error bars represent the standard deviation of three measurements. Full size image Clinical research has shown that multi-protein measurements provide more accurate diagnostic results. Biomarker development research has identified many helpful proteomics panels for disease diagnosis and prognosis, including cancer [27] , [28] , cardiovascular disease [29] , diabetes [33] , Alzheimer’s disease [34] and others [35] . For example, a four-biomarker panel has been developed for detecting early-stage ovarian cancer, and an 18-protein panel is used for the diagnosis of early Alzheimer’s disease [27] , [34] . Current protein-based biomarker assay methods mostly use ELISA, which serves as the clinical gold standard. In traditional ELISA methods, colorimetric, fluorescent, electrochemical or magnetic signals are introduced to transduce the binding event of a protein to a specific recognition molecule into a readout signal [7] , [8] , [9] , [10] , [36] . As advanced instrumentation is always required for quantitative detection, most of these methods are not ideal for POC applications, due to the high cost and/or complicated operation. We have created a new volumetric POC platform that allows quantitative, multiplexed and instrument-free protein measurement. The V-Chip presents an innovative combination of low cost, portability, and rapid operation and readout. Compared with other microfluidics- and nanotechnology-based methods, this device has the following merits. Affordability: our device uses two pieces of glass with microfluidics channels and primary antibodies to capture serum protein biomarkers. Glass slides are regular low-cost materials; microfabrication cost will be greatly decreased if mass production is employed; and the amount of each antibody is minimal as the spot size is miniaturized. Ease of operation: sample loading is as simple as traditional ELISA and measurement only requires a slide of the glass plates. Minimum requirement for accessories: only a 1-ml syringe is required to load blood/serum samples into the V-Chip at the current stage. In the future, an automated blood handling kit will be included with the V-Chip assay. Portability: the platform is 75 × 50 mm in size and less than 20 g in total weight. Multiplexing: the V-Chip is capable of measuring up to 50 tests simultaneously. Sensitivity and dynamic range: the V-Chip has been proven to be competitive with the pregnancy hCG-test in our preliminary test. Easy readout and quantitation: reading the advancement of the bars will provide quantitative and visualized data. Simple integration with telemedicine and cloud medicine: the bar chart could be captured as an image using a smart phone, similar to a barcode reader and transmitted to a cloud computer for instant medical suggestions in the future. Photolithography All devices were designed as computer graphics using AutoCAD software and then printed out as transparency photomasks by CAD/Art Services Inc. (Bandon, OR) with resolution at 10 μm. Fabrication of the V-Chip device used the standard lithography process, as shown in Supplementary Fig. S1 . The glass slides (75 × 50 × 1 mm, Corning Inc.) were first spin-coated with a 10-μm-thick layer of SPR220-7 photoresist (MicroChem Corp.). The glass slides were dried by baking at 75 °C for 3 min and 115 °C for 5 min to promote resistance to adhesion. After cooling to room temperature, the glass slides with the photoresist coating were aligned with a photomask containing the designed wells and channels. The photomask and glass slides were exposed to ultraviolet light for 50 s. Then the photomask was removed from the glass slide and the glass slide was developed by immersing in SPR developer solution (MF-CD26, MicroChem Corp.) for 3 min. During this step, only the exposed areas were dissolved in the solution. The slides were thoroughly rinsed with Millipore water and dried with nitrogen gas. Glass etching and preparation of loading holes Before glass etching, the back of the glass slide was covered with polyvinyl chloride sealing tape (3 M) to protect from etching. The taped glass slides were then carefully immersed in a plastic container with a glass etchant (1:0.5:0.75 mol l −1 HF/NH 4 F/HNO 3 ) to etch the photolithography pattern [15] , [16] . A 35 °C constant-temperature water bath was used to control etching speed. At the etching time (45 min), wells and channels were etched into the glass slides with the depth of ~50 μm. After that, the tape was peeled off and the slides were thoroughly rinsed with acetone and isopropanol to remove the photoresist. Access holes were prepared with a diamond drill (0.031 inch in diameter, Harvey Tool). Surface hydrophobic modification For surface modification, the glass slides were acid-cleaned in piranha solution (H 2 SO 4 :H 2 O 2 =7:3) for 1 h and rinsed with Millipore water. After being subjected to an oxygen plasma treatment, the glass slides were given a hydrophobic coating by silanizing with tridecafluoro-1,1,2,2-tetrahydrooctyl-1-trichlorosilane (Pfaltz and Bauer, Inc.) [15] , [16] . The glass plates were baked at 120 °C for 30 min, rinsed with isopropanol and Millipore water, and dried with nitrogen gas. Capture antibody immobilization The wells were cleaned by applying drops of piranha solution for 1 h, then rinsed with Millipore water and dried with nitrogen gas. After that, 10% (3-glycidoxypropyl) trimethoxysilane (GPS, Sigma) in toluene was added into each well using a pipette. The solution was kept in each well for 30 min, and then rinsed with fresh toluene to remove extra GPS molecules. Then the glass slides were dried using dry nitrogen gas and baked at 120 °C for 30 min. Epoxy groups were covalently modified onto the surface in each well [20] . Capture antibodies were covalently immobilized in the ELISA wells by reaction with the epoxy group on the glass surface. The capture antibodies were carefully added into each well and incubated at 4 °C overnight. Then the wells were washed with 5% bovine serum albumin (BSA, Sigma) several times to avoid nonspecific binding. Assembly and operation of the V-Chip Five microlitres of Fluorinert liquid FC-70 (Hampton Research) were added to the top device plate with the patterns facing up and a blank glass slide was pressed down on it to spread the oil. After the oil was completely spread, the blank glass slide was removed and the device slide was spun at 2000, r.p.m. for 20 s to remove the excess FC-70. Then the top device plate was assembled with the bottom plate and an ultrathin FC-70 oil layer was formed between the two glass slides ( Supplementary Movie 1 , Supplementary Figs S1 and S2 ). The oil layer served as a lubricant and to render the device airtight. The wells on the top plate were positioned to partially overlap with the wells on the bottom plate, forming a continuous ‘N’-shaped fluidic path in the horizontal direction. To load a solution into the V-Chip, a pipette tip containing the sample or reagent was inserted into the left inlet of the fluidic path in the assembled device. The solution was loaded into the wells by pushing the pipette manually. To obtain the readout, the top plate was slid as shown in Supplementary Movie 1 to change the flow direction from horizontal to vertical. V-Chip ELISA reaction For the detection of hCG, magnetic beads (Dynabeads M-270 epoxy, 2.8 μM, Invitrogen) conjugated with capture antibodies were loaded into the ELISA chamber and immobilized by a magnet. Subsequently, different concentrations of hCG (Abcam) solution (0, 2, 5, 10, 10 2 , 10 3 , 10 4 and 10 5 mIU in phosphate-buffered saline (PBS) buffer, pH 7.4) were loaded and incubated at room temperature for 30 min. The chamber was then washed with washing solution (2% BSA and 0.05% Tween-20 in PBS buffer) three times. Afterwards, the catalase probe was added through the inlet, incubated for another 30 min, and washed four times with washing solution and once with PBS buffer. The ELISA readout was obtained by sliding the V-Chip to allow the catalase probe to make contact with hydrogen peroxide. For the cell lysate assays, the wells of the assembled V-Chip were coated with capture antibodies, and washed with 2% BSA twice. Then 10 μl of the cell lysate was continuously loaded into the wells through the left inlet holes and the loading step was repeated four times. At the final step, the chip was incubated at room temperature for 1 h and washed with washing solution (2% BSA and 0.05% Tween-20 in PBS buffer) three times. Following this, the catalase probe was added through the inlet and incubated for a further 1 h. The chamber was washed four times using washing solution and once with PBS buffer. The patient sera were collected under the protocol IRB0412-0066 approved by the institutional review board of the Methodist Hospital Research Institute. One microlitre of each serum sample was carefully added to each ELISA well with a pipette, and incubated at room temperature for 1 h. The wells were then washed with washing solution (2% BSA and 0.05% Tween-20 in PBS buffer) three times. Subsequently, the top slide, coated with FC-70, was placed onto the bottom glass slide. The ELISA fluidic path was washed with 2% BSA twice. The catalase probe was added through the inlet and incubated for a further 1 h. The wells were then washed four times with washing solution and once with PBS buffer. For future multiplexed serum biomarker assays, the serum sample can be directly applied to the V-Chip ELISA channel, and all proteins of interest can be quantitated in a single assay without the need for additional instrumentation, similar to the cell lysate assay shown above. Ink and H 2 O 2 loading Twenty microlitres of red ink and 0.45 M H 2 O 2 were loaded into their respective fluidic paths from the left inlet. The solution filled the fluidic path because of the hydrophilic interaction between the solution and the glass surface in the fluidic path. Readout After the completion of the ELISA reaction and reagent loading, the V-Chip was carefully slid by moving the top slide at an oblique angle. As a result, the wells on the top and bottom slides formed a ‘Z’-shaped fluidic path in the vertical direction. The red ink was pushed into the small channels and the inked bands moved into the channels due to the oxygen pressure generated ( Supplementary Movie 1 , Fig. 1 and Supplementary S3 ). The results were recorded with a camera and the frontiers of ink advancement were marked for quantitation. How to cite this article: Song, Y. et al. Multiplexed volumetric bar-chart chip for point-of-care diagnostics. Nat. Commun. 3:1283 doi: 10.1038/ncomms2292 (2012).